Revisiting the identification ofSyllipsimopodi bideniand timing of the decabrachian-octobrachian divergence 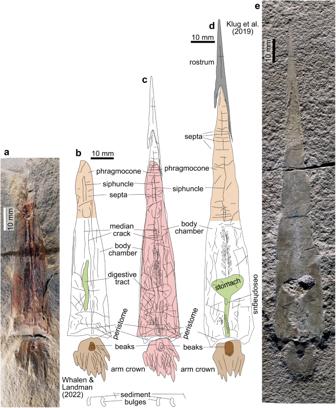Fig. 1: The early coleoidsGordoniconus beargulchensisandSyllipsimopodi bidenifrom the Bear Gulch Limestone, Heath Fm., Serpukhovian, Fergus County, Montana, USA. Light brown—phragmocone; middle brown—arm crown; dark brown—buccal mass; green—digestive tract; middle grey—rostrum.aPhoto of the holotype ofS. bideni(increased contrast after1: suppl. fig. 6), ROMIP 64897.bLine drawing aftera.cOverlay ofb(filled in pink) andd(scaled down by about 20% to fit body chamber width).dLine drawing aftere.eHolotype ofG. beargulchensis, AMNH 50267; photo modified after10b. We compared the holotypes of the two coleoids by tracing visible structures in published photos. First, we gently enhanced the contrast using the raster graphics editor Adobe PhotoShop CS6. We saved the photos as single-layer tif-files and imported them into the vector graphic software CorelDraw X8. There, we traced all visible structures independent of their meaning. Subsequently, we homologized those structures displaying sufficient detail. Finally, we overlaid those drawings by adapting their scales to each other to demonstrate the great degree of morphological similarity. Reporting summary Further information on research design is available in the Nature Portfolio Reporting Summary linked to this article.